Dirac leaky-wave antennas for continuous beam scanning from photonic crystals Leaky-Wave Antennas (LWAs) enable directive and scannable radiation patterns, which are highly desirable attributes at terahertz, infrared and optical frequencies. However, a LWA is generally incapable of continuous beam scanning through broadside, due to an open stopband in its dispersion characteristic. This issue is yet to be addressed at frequencies beyond microwaves, mainly as existing microwave solutions (for example, transmission line metamaterials) are unavailable at these higher frequencies. Here we report leaky-wave radiation from the interface of a photonic crystal (PC) with a Dirac-type dispersion and air. The resulting Dirac LWA (DLWA) can radiate at broadside, chiefly owing to the closed Γ-point bandgap of the Dirac PC. Thus, the DLWA can continuously scan a directive beam over a wide range of angles by varying the frequency. These DLWAs can be designed at microwave as well as terahertz to optical frequencies, with feasible dimensions and low losses. Zero-index metamaterials (ZIMs), including epsilon-near-zero (ENZ) metamaterials [2] , offer unique and fascinating wave phenomena such as tunnelling of waves through channels and bends [3] , [4] , tailoring the phase of the radiation patterns from arbitrary sources [5] , directive emission of sources [6] , [7] and unusual bending of light for extremely short focusing [8] , to name a few. It is also possible to enhance and shape the air-side radiation patterns of radiators by placing them on (an)isotropic ENZs and ZIMs [9] . It has even been proposed that ENZs can enable electric levitation of a dipole [10] . The directive emission (gain enhancement) using bulk ZIMs, as well as the atypical bending of light using ZIMs [8] , are primarily owing to Snell’s law. Air has a higher refractive index than the ZIM, hence the angle of refraction in air is smaller than in the ZIM, contrary to typical dielectrics. If a radiator is embedded inside the ZIM, the waves exiting the ZIM are collimated, causing a highly directive beam. Leaky waves [11] , [12] , [13] can also play a significant role in directive emission from finite ZIMs [14] , [15] . Leaky-wave radiation involves gradual leakage of electromagnetic energy over a structure, most commonly utilized in the context of Leaky-Wave Antennas (LWAs). This simple gradual leakage of energy enables radiation of highly directive and narrow beams from the antenna. LWAs are also capable of scanning the beam direction by simply changing the frequency of operation. LWAs have been traditionally used and extensively studied at microwaves [11] , [12] , [13] . But these structures offer capabilities that also make them excellent candidates for new frontiers in the terahertz, infrared and even optical applications [16] . The radiation of a unidirectional leaky wave towards broadside has been a challenging and elusive concept. Continuous leaky structures such as slot waveguides are only capable of forward scanning above the cut-off (broadside) of the leaky mode [11] . Periodically perturbed waveguides, such as periodically loaded dielectric waveguides [16] , [17] are capable of both forward and backward scanning away from broadside, but typically have an open stopband around broadside due to mode coupling [11] , [18] . Hence, such structures so far could never achieve true broadside radiation and could only radiate ‘close’ to broadside [11] . Consequently, these structures are typically mismatched at their input terminals around broadside frequencies. By centre feeding a leaky structure, it is possible to produce a single broadside beam from the two opposing beams leaking from the two sides of the feed [19] . However, this beam quickly splits into two halves as the frequency changes, preventing a scanning operation. Moreover, a typical side-fed (unilateral) excitation of these LWAs (and other typical leaky structures) can never achieve true broadside radiation. It was demonstrated at microwaves that the stopband can be closed in transmission-line metamaterial LWAs, by ‘balancing’ the shunt and series transmission line impedances [20] , [21] , [22] , [23] . Such antennae can be simply identified as transmission lines with sub-wavelength unit cells having both series and shunt lossy resonators. When the two resonant frequencies are made equal, a closed stopband situation arises. In addition, the existence of both series and shunt radiation resistances that have a specific ratio in the unit cell is a necessary condition to achieve actual broadside radiation even under the balanced condition [22] . Elimination of the open stopband in one-dimensional (1D) periodic printed LWAs at microwaves was demonstrated in ref. 23 , using a stub-matching technique in the unit cell. These concepts have so far been demonstrated only at microwaves. Primarily this is because they are either applicable to periodic structures with a very sub-wavelength unit cell period ( ) such as transverse electromagnetic (TEM) and quasi-TEM mode (mainly microstrip type) LWAs, or require situations where it is possible to realize printed circuit or stub elements, or more complicated unit cells with additional mechanisms [23] , [24] , and/or situations where it is appropriate to apply transmission-line modelling as in refs 19 , 20 , 21 , 22 to determine the balanced condition and close the stopband. To date, however, neither a dielectric LWA that has a closed broadside stopband been proposed, nor has a LWA been demonstrated based on a photonic crystal (PC) that is devoid of a Γ-point bandgap, and satisfies the appropriate radiation mechanisms (similar to ref. 21 ), to enable true unilateral broadside radiation and continuous beam scanning. Such structures are extremely useful for reliable leaky-wave operation, especially at higher frequencies beyond microwaves. Some dielectric based and optical LWAs have been reported thus far in the literature [16] , [17] , [25] , [26] , which, however, all suffer from the broadside open stopband issue. Recently the study by Huang et al . [4] reported a remarkable discovery of an effective zero-index behaviour in PCs. This zero-index PC is a typical 2D PC operating in a regime where two inverted Dirac dispersion cones meet ‘at the Γ-point’ of the PC, due to an accidental degeneracy of modes. Reference [4] showed that this leads to an effective zero-index behaviour around the Γ-point, and verified this by effective medium theory beyond the long wavelength limit [27] . Based on the work of Huang et al . [3] , Moitra et al . [6] recently demonstrated the all-dielectric zero-index PC for directive emission of point sources at infrared frequencies. In this work, we utilize the Dirac-type PC of ref. 3 and ref. 6 to demonstrate that these structures can be made to radiate to realize directive Dirac LWAs (DLWAs). The proposed class of DLWAs has an important advantage over common LWAs as they are capable of radiating through broadside as the directive beam is scanned by varying the frequency. The DLWA has a closed stopband, matched response, non-fluctuating leakage constant and real non-zero Bloch impedance at and around broadside. This is achieved by utilizing the Dirac-type dispersion of the PC at the Γ-point, as well as appropriate shunt and series radiation mechanisms in the unit cell. The DLWA is also capable to steer or scan the directive beam over a wide range of angles off broadside (in both forward and backward directions) simply by changing the frequency, with a matched response. These DLWAs can open doors for continuous and reliable leaky-wave operation at microwave to terahertz and optical wavelengths. Exploiting the Dirac dispersion for leaky-wave radiation The dispersion characteristics of the 2D Dirac PC of ref. 3 offer some unique features. As shown in Fig. 1a , there are two inverted dispersion cones (Dirac cones) touching at a single Dirac point ( f D ). Moreover, the PC is designed such that this Dirac point occurs at the Γ-point ( k x = k y =0). The dispersion bands on either Dirac cones have a linear change in frequency when traversing the Γ− X path on the Brillouin zone near the Dirac point. The continuous and linear dispersion curves are actually the characteristic feature of the Dirac point [4] . Each band is shown in ref. 3 to comprise an electric monopole and a transverse magnetic dipole. At frequencies just about the Dirac point, the medium behaves as an effective zero-index media in an almost isotropic manner as shown in Fig. 1b . Such effective zero-index behaviour was verified in ref. 3 using effective medium theory beyond the long wavelength limit [27] . Therefore the PC supports a propagation that has a gradual change in the transverse wavenumber as the frequency changes, including the Γ-point. This Dirac-type dispersion behaviour also implies that the PC has a closed bandgap at the Γ-point at a particular frequency f D , as a result of the two inverted and touching dispersion cones. 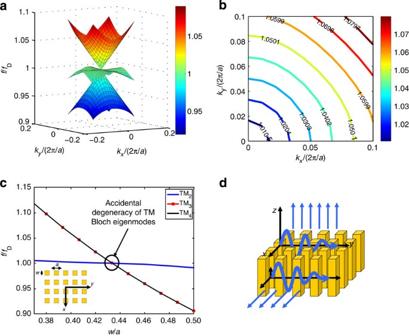Figure 1: Exploiting a photonic crystal with a Dirac-type dispersion for leaky wave radiation. (a) Two inverted Dirac dispersion cones touching at the Γ-point of the Brillouin zone, showing a closed bandgap in a two-dimensional (2D) Dirac-type photonic crystal (PC). (b) Iso-frequency contours above the Dirac point, showing an isotropic zero-index behaviour in the PC. (c) Mode chart of the three eigenmodes at the Γ-point around the accidental degeneracy dimensions for the 2D Dirac PC. Inset shows the periodic arrangement of the PC. (d) The Dirac photonic crystal with an interface to air for leaky-wave radiation. The dispersion diagrams and mode chart results are for a Dirac PC based on the work of Huanget al.4 Figure 1: Exploiting a photonic crystal with a Dirac-type dispersion for leaky wave radiation. ( a ) Two inverted Dirac dispersion cones touching at the Γ-point of the Brillouin zone, showing a closed bandgap in a two-dimensional (2D) Dirac-type photonic crystal (PC). ( b ) Iso-frequency contours above the Dirac point, showing an isotropic zero-index behaviour in the PC. ( c ) Mode chart of the three eigenmodes at the Γ-point around the accidental degeneracy dimensions for the 2D Dirac PC. Inset shows the periodic arrangement of the PC. ( d ) The Dirac photonic crystal with an interface to air for leaky-wave radiation. The dispersion diagrams and mode chart results are for a Dirac PC based on the work of Huang et al . [4] Full size image It was found in ref. 3 that the Dirac point can occur at the Γ-point as a result of an ‘accidental degeneracy’ of modes in the PC. Accidental degeneracy of eigenmodes can occur both in dielectric resonators [28] and in dielectric PCs [4] . In accidental degeneracy, multiple orthogonal eigenmodes of a structure become degenerate (resonate at the same frequency), but this degeneracy is ‘accidental’ as it is not due to symmetry of the structure or lattice. Such a multi-resonant effect typically occurs at a certain set of dimensions given the boundary conditions. Accidental degeneracy of 3D resonant modes of a typical cylindrical (puck-shaped) and half-cut dielectric resonator was previously demonstrated in ref. 27 to realize quadruple-mode and dual-mode dielectric resonators. At the degenerate point, a single physical cylinder was shown to sustain four orthogonal eigenmodes at the same frequency. This allowed the development of ‘single cavity four-pole’ filters, offering a significant size reduction [28] . The accidental degeneracy of Bloch eigenmodes in the PC of ref. 3 can be simply seen with the trend in the resonance frequencies of the allowable Bloch eigenmodes with respect to a change in a critical geometrical dimension. This is best exemplified through the mode chart as shown in Fig. 1c for the unit cell of the 2D Dirac PC of ref. 3 and ref. 6 , similarly to what was previously shown for modes of a dielectric resonator in a metallic cavity [28] . The PC is composed of periodic posts or rods with a square cross-section of side ‘ w ’ and high permittivity (for example, Si, ε r =13.7), arranged in a lattice with period ‘ a ’ inside a lower permittivity host medium (for example, SiO 2 , ε r =2.1) as depicted in the inset of Fig. 1c . At a specific fill factor of the dense dielectric ( w / a ), three TM n Bloch modes (a pair of symmetrically degenerate modes and a third mode) accidentally degenerate and resonate at the same Dirac frequency ( f D ), for the Γ-point boundary conditions applied to the unit cell. Due to their orthogonality, the modes do not couple and can coexist at the same frequency at the degenerate point. The central idea here is that at the interface of such a PC with air, like the one shown in Fig. 1d , a leaky mode may be supported of which its propagation constant is dependent on frequency. More importantly, the propagation can exist even at the Γ-point with no frequency gap. Note that a bandgap at the Γ-point of a leaky PC is equivalent to the open broadside stopband in 1D LWAs. Therefore, we can achieve backward and forward, as well as broadside (at the Dirac point) leaky radiation from the interface of a PC with such Dirac dispersion behaviour, resulting in the DLWA. The resulting DLWA can also be matched at the Γ-point as there is no stopband and it also has both of the necessary shunt and series radiation resistances in the lossy resonator model of the unit cell, as will be discussed later. The leaky Dirac PC In order for the PC to couple to propagating waves in air, we need to create an interface between the PC and air. Depending on the scenario, one could envision different mechanisms for creating a leaky interface. Let us consider the unit cell of the top perforated leaky Dirac PC for 2D propagation in Fig. 2a and for 1D propagation in Fig. 2b . The unit cells are made of a high permittivity dielectric rod inside a low permittivity host medium in both cases. To enforce the electric field to lie along the z -axis, the rod and host are placed between two parallel perfect electric conductors (PEC). 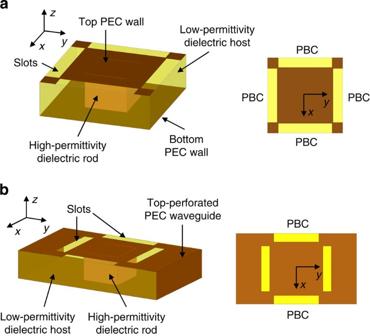Figure 2: A leaky Dirac photonic crystal. Unit Cell of the (a) two-dimensional (2D) Dirac photonic crystal (PC) and (b) one-dimensional (1D) Dirac PC with top perforations realized with slots in the metal waveguide. Inb, the periodicity is in thex-direction, and Perfect Electric Conductor walls terminate the cell in the y-direction (as opposed to being periodic as ina). Figure 2: A leaky Dirac photonic crystal. Unit Cell of the ( a ) two-dimensional (2D) Dirac photonic crystal (PC) and ( b ) one-dimensional (1D) Dirac PC with top perforations realized with slots in the metal waveguide. In b , the periodicity is in the x -direction, and Perfect Electric Conductor walls terminate the cell in the y-direction (as opposed to being periodic as in a ). Full size image The 2D PC case therefore resembles a dielectric-filled, Parallel-Plate Waveguide (PPW). As the 2D PC is infinitely periodic in the x − y plane, the opposing sides of the cell are covered with periodic boundaries to enforce a Floquet periodicity of ( k x , k y ) between them. The 1D PC is similarly periodic in the x -direction, but in the transverse direction ( y -direction) the cell is terminated with PEC walls. This turns the unit cell into a section of a dielectric-loaded rectangular waveguide. The top PEC plate is then perforated to allow the leakage of fields outside the guides. In the 2D leaky case, simulations reveal that the three TM n Bloch modes of the Dirac PC (as discussed earlier and reported in Fig. 1c ) are established between the parallel plates. These three modes can be made degenerate (with appropriate adjustment of the dimensions) at the Γ-point to establish the touching Dirac dispersion cones for 2D propagation. Two of these three modes are actually dual degenerate (as shown in Fig. 1c ) due to symmetry. In the 1D leaky case, eigenmode simulation shows that only two Bloch eigenmodes are established inside the waveguide section given that the periodic boundary condition is established between the two ends of the guide, around the frequency of interest. The two modes can again be made degenerate at the Γ-point of the Brioullin zone with the appropriate dimensions of the post. These are two of the original three TM n Bloch modes of the Dirac PC. In the 1D leaky case, we are only dealing with 1D propagation, and only two TM n Bloch modes are required to become degenerate to achieve a Dirac-type dispersion behaviour. One of the symmetric dual-degenerate modes from the 2D propagation case is not used in the 1D propagation. The 1D leaky Dirac PC unit cell is designed as described in the Methods section. The two Bloch modes of the 1D leaky case are shown in Fig. 3a , where they are both degenerate at the Γ-point of the Brioullin zone at f D , that is, at k x =0, which leads to a 1D Dirac-type dispersion for the PC. These two Bloch eigenmodes are orthogonal by definition for the given boundary conditions. The similarly sized slots are designed such that the modes also have a finite (due to radiation) and comparable quality factors Q , which is a representation of the radiation of the modes and the leakage constant. The design procedure of the cell is explained in the Methods section. 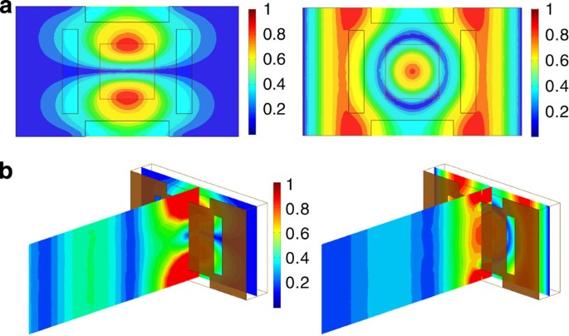Figure 3: Accidental degeneracy of two eigenmodes in the leaky Dirac PC at the Γ-point. (a) Normalized E-field magnitude in thex–yplane for the two eigenmodes of interest at the Γ-point frequency of the one-dimensional (1D) Dirac PC. (b) Normalized |Real{E}| in thex–zplane for the two leaky eigenmodes at the Γ-point frequency. Figure 3: Accidental degeneracy of two eigenmodes in the leaky Dirac PC at the Γ-point. ( a ) Normalized E-field magnitude in the x – y plane for the two eigenmodes of interest at the Γ-point frequency of the one-dimensional (1D) Dirac PC. ( b ) Normalized | Real { E }| in the x – z plane for the two leaky eigenmodes at the Γ-point frequency. Full size image Any field that exists outside the guide must also meet these boundary conditions at the unit cell walls. If the eigenmode is radiating, then propagating waves outside the guide in air would propagate away from the top surface of the guide. This is shown graphically in Fig. 3b with the magnitude of the real part of the electric field outside the unit cell. The figure depicts propagating waves emanating away from the top surface for the two radiating eigenmodes. The perforations in the top metal allow for coupling of the mode(s) inside the parallel-plate walls to spatial modes outside. The perforations are placed such that the overall configurations still support the original triple (2D) and double (1D) modes of the guide. The perforations can be in the form of different shapes such as circular or square, placed at appropriate edges of the unit cell. It should be noted that by creating the top perforations in the guide, the original Dirac point of the unperforated PC breaks up and shifts in frequency, that is, the accidental degeneracy of the new crystal differs from the original PC in a non-perforated waveguide (a similar remark applies to the 2D case). Therefore, we adjust the filling ratio of the dielectric to achieve another degenerate point, and adjust the period to account for the frequency shift, using the open eigenmode simulations described in the Methods section. The DLWA The proposed 1D Dirac-type LWA is shown in Fig. 4 with the 3D (a), top (b) and front cross-section (c) views. This antenna is made directly from cascading the leaky Dirac PC unit cell that was described previously and shown in Fig. 2b . The design of the antenna therefore mainly simplifies to designing the appropriately tuned leaky unit cell as explained in the Methods section. The cross-section of the antenna (in the y – z plane) is simply the metallic rectangular waveguide filled with the host dielectric and loaded with one high permittivity rod. The length of the antenna (in the x -direction) has enough cells to radiate a desired amount of input power (typically >90% in LWAs). The structure is fed from one of its ends and can be either terminated at the other end with a matched load (as done here) or left open. Further information on the configuration of the DLWA is described in the Methods section. 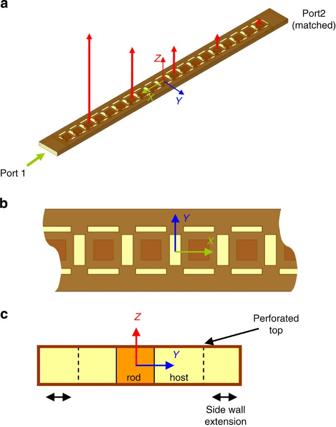Figure 4: A 1D DLWA. (a) Three-dimensional view and (b) top view of the 19-cell DLWA made from cascading the unit cells of the leaky Dirac Photonic Crystal (PC). Unilateral excitation of the antenna from port 1. Residual power is collected at port 2, which is matched to the leaky structure. Port 2 can be left open in long antenna where all power is radiated. (c) Cross-section of the antenna, showing placement of the high permittivity rods and sidewall extension. Figure 4: A 1D DLWA. ( a ) Three-dimensional view and ( b ) top view of the 19-cell DLWA made from cascading the unit cells of the leaky Dirac Photonic Crystal (PC). Unilateral excitation of the antenna from port 1. Residual power is collected at port 2, which is matched to the leaky structure. Port 2 can be left open in long antenna where all power is radiated. ( c ) Cross-section of the antenna, showing placement of the high permittivity rods and sidewall extension. Full size image The S-parameters of the DLWA are reported in Fig. 5 around the Γ-point, showing a remarkable performance in the context of existing LWA literature. We can see that the antenna is perfectly matched (| S 11 |<−20 dB) for frequencies at and close to the Γ-point of the PC, that is, all of the incident power is accepted. The low transmission to port 2 (| S 21 |<−10 dB) also indicates that very little portion of the input power remains at the end of the antenna (almost all of the incident power is radiated out). The simulated structure is assumed to be lossless (aside from radiation), although losses can be accounted for as discussed later. 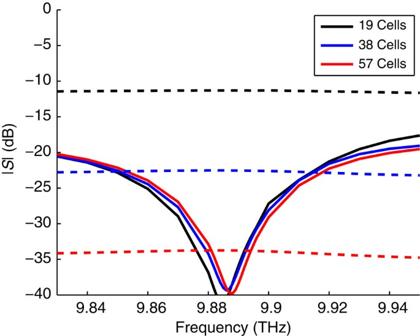Figure 5: Perfect matching of the DLWA around broadside. S-parameters of the DLWA for three antenna lengths close to broadside (solid lines areS11and dashed lines areS21). Perfect matching (|S11|→0) shows a closed bandgap at the Γ-point, as well as close to zero transmission (|S21|→0) shows complete radiation of power for all lengths. Figure 5: Perfect matching of the DLWA around broadside. S-parameters of the DLWA for three antenna lengths close to broadside (solid lines are S 11 and dashed lines are S 21 ). Perfect matching (| S 11 |→0) shows a closed bandgap at the Γ-point, as well as close to zero transmission (| S 21 |→0) shows complete radiation of power for all lengths. Full size image This dipping trend of | S 11 | of the DLWA is a behaviour completely opposite to that of typical periodic LWAs with a broadside stopband. Periodic LWAs typically have a rise in | S 11 | near the broadside frequency (referred to as increased voltage standing wave ratio) [11] , [24] , which becomes more serious with increasing the antenna length (the closer they approach to the infinitely periodic case). This is definitely not the case here and hence this is one of the indications that the DLWA is markedly different. Radiation characteristics The radiation pattern of the DLWA is reported in Fig. 6a , for the principal φ =0° plane, showing a directive beam pointing exactly at broadside. A gain of 14.1 dB is attained exactly at broadside for this 19-cell example. Note that all reported gain values are essentially ‘realized gain’ values, as the antenna is fully matched, as was shown in Fig. 5 . 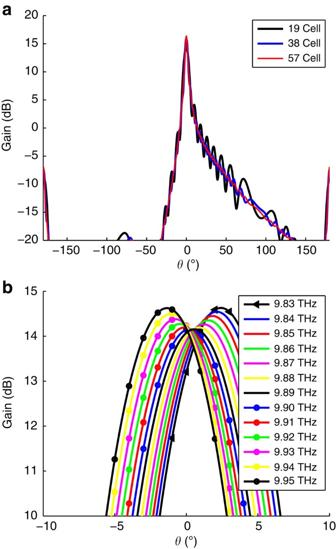Figure 6: Directive broadside radiation of the DLWA. Gain plot of the broadside beam in theφ=0° plane for three different antenna lengths (a). Figure shows broadside radiation is in fact occurring due to a true leaky wave and is not due to finite antenna effects. As the length of antenna is increased, the gain increases and the pattern ripples are removed. (b) Radiation around broadside for the 19-cell DLWA, in theφ=0° plane. Figure 6: Directive broadside radiation of the DLWA. Gain plot of the broadside beam in the φ =0° plane for three different antenna lengths ( a ). Figure shows broadside radiation is in fact occurring due to a true leaky wave and is not due to finite antenna effects. As the length of antenna is increased, the gain increases and the pattern ripples are removed. ( b ) Radiation around broadside for the 19-cell DLWA, in the φ =0° plane. Full size image The broadside radiation can also be interpreted from a zero-index perspective. In fact, our DLWA is in effect a waveguide filled with an effective zero-index medium (see Supplementary Note 1 and Supplementary Fig. 1 ), such that the phase progression of fields along the surface and at the edges of each unit cell is zero, leading to in-phase radiating elements (see Supplementary Fig. 2 ) and broadside radiation. These two viewpoints are equivalent and converge to the same effect. As the frequency is changed about the broadside frequency, the beam direction varies as shown in Fig. 6b . The beam is highly directive with negligible variation in directivity around broadside, which can in fact be further mitigated in refined designs. This shows that the antenna can sweep a beam from the forward direction through broadside, and to the backward direction, and vice versa by changing the frequency, without any detriment to any of the antenna performance metrics or gaps in radiation. The sidelobe levels are low and in fact there is only one main beam with ripples on the pattern due to the finite length of the antenna simulated (an infinite structure would not have any ripples). The 3D gain plots of the DLWA are shown in Fig. 7 , which demonstrate the directive fan-beam nature of the pattern as expected from a 1D leaky structure. The results pertaining to longer antennae confirm that the DLWA indeed has a closed broadside stopband, as the antenna becomes longer. The S-parameters in Fig. 5 show that all power is again accepted (dipping S 11 ) and more power is radiated (lower S 21 ) as the antenna length is increased. The gain of the broadside beam also increases to 16.4 dB, and the pattern ripples are almost completely removed with no sidelobes, as the length of the DLWA is increased from 19 to 57 cells, as seen in Fig. 6a . This further confirms that broadside radiation is in fact occurring due to a true leaky wave and is not due to finite-LWA effects. 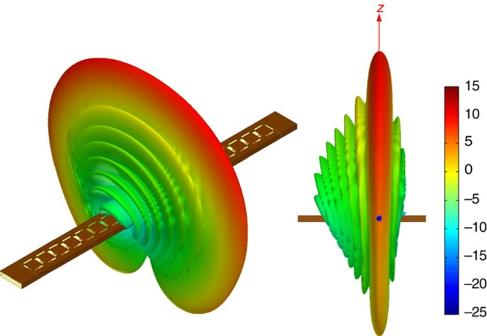Figure 7: Three-dimensional radiation pattern of the DLWA. Gain of the 19-cell DLWA (in a 40-dB scale range), showing a narrow fan beam pointing right at broadside. Figure 7: Three-dimensional radiation pattern of the DLWA. Gain of the 19-cell DLWA (in a 40-dB scale range), showing a narrow fan beam pointing right at broadside. Full size image It is emphasized that the resulting DLWA does not experience mode coupling/cancellation at the Γ-point, contrary to typical LWAs. Rather, it utilizes the orthogonal degenerate Bloch TM eigenmodes of the PC and directly establishes fast waves at its interface with air. The accidental degeneracy guarantees a closed bandgap in the dispersion diagram of the resulting PC. We make the connection here that a Dirac-type dispersion behaviour is equivalent to the closed stopband condition in metamaterial transmission lines [21] , and along with the shunt+series radiative losses (see Supplementary Methods ) leads to the true broadside leaky-wave radiation from the PC. Leaky-wave parameters The extracted dispersion diagram of the antenna is shown in Fig. 8 for frequencies close to the Γ-point. It can be seen that there is no stopband and the dispersion curve continuously links the backward region to the forward region without any gap or change in the linear trend. Moreover, the group velocity is not zero at broadside (the tangent to the curve does not have a zero slope), confirming that broadside radiation is indeed possible. 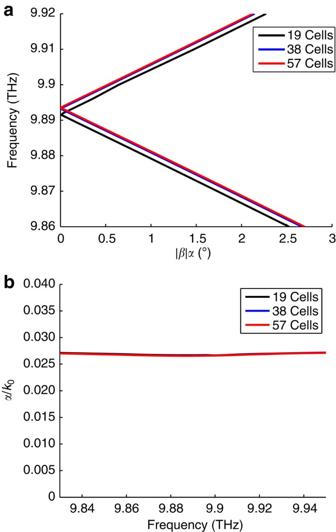Figure 8: Propagation constant of the DLWA. (a) The extracted dispersion diagram from the N-cell simulation, showing a closed broadside stopband. (b) The normalized attenuation (leakage) constant (α/k0) around broadside frequencies, showing almost no variation. Figure 8: Propagation constant of the DLWA. ( a ) The extracted dispersion diagram from the N-cell simulation, showing a closed broadside stopband. ( b ) The normalized attenuation (leakage) constant ( α / k 0 ) around broadside frequencies, showing almost no variation. Full size image The attenuation (leakage) constant α and phase constant β were obtained using S-parameter retrieval from the driven N-cell simulations described in the Supplementary Methods . It is found that at f D =9.892 THz, β =0 which is the Γ-point or the Dirac degeneracy frequency. The leakage constant shown in Fig. 8b is found to be α / k 0 =0.0267 at f D . The figure also depicts how the leakage constant does not vary close to the Γ-point, contrary to typical LWAs. Various effects such as an open stopband or not supporting the appropriate radiation mechanisms typically manifest themselves with abrupt variations in the leakage constant around broadside in LWAs [22] . The size of the perforations provides a control mechanism to tailor the leakage factor. Adjustment of the perforation size is done with the appropriate minor adjustments of the filling ratio and/or period to ensure that the degeneracy point (closed stopband) is maintained at the desired design frequency for broadside radiation. In the Supplementary Methods , the behaviour of the 1D leaky Dirac PC unit cell is modelled with a lossy series resonator and a lossy shunt resonator around the Γ-point, and is shown in Supplementary Fig. 3 and Supplementary Fig. 4 . The extracted resonances ( f se ≈ f sh ≈9.892 THz) and the fitted circuit-model parameters ( L se =1 × 10 −11 H, C se =2.5871 × 10 −17 F, R se =8.113 Ω, L sh =2.25 × 10 −13 H, C sh =1.15 × 10 −15 F, G sh =5.738 × 10 −4 S) of the unit cell show that the stopband of such a structure is indeed closed. Equally important, there exits both a series resistance and a shunt conductance (meaning both a series radiation resistance and a shunt radiation conductance) in the circuit model of the unit cell and in an appropriate ratio to ensure matching at broadside. This condition guarantees that the Bloch impedance of the periodic structure can be made real and finite at the Γ-point, with little variation over the frequency. This in fact can be seen as a necessity for correct broadside radiation of a general periodically leaky unit cell (regardless of its dimensions with respect to the wavelength) and encompasses the condition of ref. 21 for leaky metamaterial transmission lines with sub-wavelength unit cells. The Bloch impedance ( Z B ) close to broadside is shown in Fig. 9a . The shunt and series radiation element values are such that the Bloch impedance of this periodic structure around the Γ-point is 119.4 Ω (also equal to . This is very close to the characteristic impedance of the incoming waveguide (121 Ω), therefore allowing a perfect matching at broadside. The Bloch impedance is also fairly constant around the broadside frequency, enabling the consistent matching of the antenna as the beam is scanned from backward to broadside to forward direction. 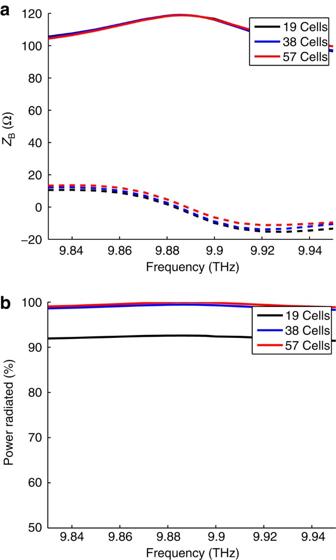Figure 9: Bloch impedance and radiation performance for different lengths of the DLWA. (a) Real (solid) and imaginary (dashed) components of the Bloch impedance of the DLWA around the Γ-point frequency extracted from the 19-cell simulation. (b) Amount of radiated power from the DLWA around broadside. Figure 9: Bloch impedance and radiation performance for different lengths of the DLWA. ( a ) Real (solid) and imaginary (dashed) components of the Bloch impedance of the DLWA around the Γ-point frequency extracted from the 19-cell simulation. ( b ) Amount of radiated power from the DLWA around broadside. Full size image The 19-cell example radiates about 93% of the incident power as typically required in LWA literature [11] , [12] , [13] . This is shown in Fig. 9b , which is the plot of the quantity 1−| S 11 | 2 −| S 21 | 2 . Longer antennae provide higher amounts of radiated power as also seen in Fig. 9b . The design of the leakage constant was done such that the DLWA had a reasonable length to radiate this much power and to be manageable for simulation purposes. Higher and lower leakage constants are also possible as mentioned earlier. Scanning ability of the DLWA Changing the frequency of operation is the most common method in LWAs to vary the angle at which the beam is pointing at [11] , [12] , [13] . Some techniques have also been proposed that enable fixed frequency scanning as in refs 28 , 29 at microwaves. The continuous scanning or steering ability of the DLWA is depicted in Fig. 10 for the leaky beam in the φ =0° plane. It can be seen that the DLWA has a wide scan range over the simulated bandwidth from 61° to −37°, when changing the frequency from 8.3 to 11.12 THz. The antenna is matched with | S 11 |<−13.5 dB over the entire range of frequencies. The gain does not vary over this frequency range and the antenna keeps its performance with about 14 to 16 dB change in peak gain. In the forward region of scanning, the transverse plane of the beam has two additional nulls in the pattern, therefore increasing the peak directivity of the beam slightly (by about 1 dB). The sidelobe levels are about −10 dB lower than each peak gain over the entire frequency range for the 19-cell example. These sidelobes are arising from pattern ripples due to finite size, and are greatly reduced by using longer antennae as was shown in Fig. 6a . 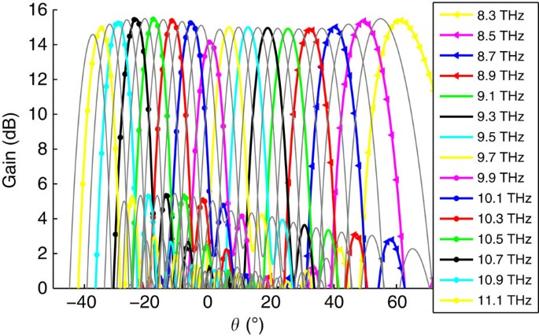Figure 10: Scanning ability of the DLWA. Changing the beam direction from backward to froward direction, through broadside by varying the frequency. The scan range is from +61° (at 8.3 THz) to −37° (at 11.12 THz). No degradation in pattern shape or beam, and with <2 dB gain variation over the wide scan range. Figure 10: Scanning ability of the DLWA. Changing the beam direction from backward to froward direction, through broadside by varying the frequency. The scan range is from +61° (at 8.3 THz) to −37° (at 11.12 THz). No degradation in pattern shape or beam, and with <2 dB gain variation over the wide scan range. Full size image The limits of the scan range are determined by the existence of other spurious modes, which can be pushed farther with refined designs. For a general LWA, the half-power beamwidth is given by Δ θ ∝ λ 0 /( L cos θ m ), where L is the total length of the antenna, θ m is the angle the beam is pointing to and λ 0 is the operating wavelength at which the beam angle is θ m (ref. 11 ). Therefore we observe slight widening of the beamwidth towards the +60° scan direction (8.3 THz), due to the shortening of the electrical length of the antenna at lower frequencies. A longer antenna with more cells has a larger electrical length at lower frequencies, and thus a narrower beamwidth is achieved at the lower frequencies of the scan range (the +60° direction). The antenna can also be made periodic in the transverse direction (by using more cells in the y -direction). This would utilize the 2D leaky PC in Fig. 2a , and again can be terminated with extended PEC walls. In addition, the proposed DLWA can be made to leak not only from the top/bottom as previously shown, but to also leak efficiently from the sides by opening the sidewalls (instead of the closed sidewalls of the waveguide situation). It is interesting to note that an open end of a PPW does not radiate significantly, however, the open end of the PPW filled with the Dirac PC can leak power quite efficiently. Supplementary Fig. 5 shows 3D directivity plots for a hybrid, side- and top-leaky structures, realized with 4 cells in the transverse direction and 20 cells in the x -direction. It can be seen that the fan beam now has peaks at φ =0° (due to top leakage) as well as φ =±90° due to the side leakage. Last, it must be noted that a 2D leaky Dirac PC can be used to realize sharp pencil beams radiating right at broadside, by exciting an N × N-cell array of the DLWA, either from the centre, side or corner. Losses At microwave frequencies, metallic waveguides have minimal conductor losses compared with any other printed-circuit technology such as printed TEM structures. Therefore, the DLWA has better loss performance compared with microstrip- or planar-type implementations as it is based on a rectangular waveguide. Moreover, it does not use sub-wavelength traces and elements, which cause significant loss. Hence, the losses at microwaves are of little concern for this design, and the antenna provides a great deal of flexibility for designing various leakage constants for the desired amount of gain, at various microwave frequencies. At optical frequencies, metal losses are of higher concern, as well as dispersive effects of metals causing them to behave as non-metals. A dispersive model (such as Drude model) for the actual metal must be used to characterize the losses at optical frequencies. At low terahertz, however, it is generally adequate to model the metal losses with the skin effect. For the 19-cell example shown here using the finite conductivity boundary condition in Ansoft HFSS and Aluminium having a DC conductivity of 3.8 × 10 7 S m −1 and Copper with DC conductivity of 5.8 × 10 8 Sm −1 , the antenna still radiates with a sharp pattern and peak gains of 8.6 dB and 9.3 dB at broadside, respectively. The antenna efficiency is about 41% for the case with Aluminium walls and 46% for the case with Copper walls. Reference [31] shows that the skin effect model used along with the ‘finite boundary condition’ in Ansoft’s HFSS simulator may even overestimate the losses in a metal rectangular waveguide in the low terahertz frequencies. Therefore our simulations are a safe estimate of the deteriorating effects due to metal losses. This suggests that a lossy implementation of the DLWA with metals at terahertz frequencies can yield perfectly usable gain levels and performance. As metal losses are higher for infrared and optical frequencies, it is more desirable to design the antenna with a metal-free slab of the Dirac PC and utilize leaky-wave radiation from its interfaces with air, similar to what was shown in Fig. 1d . This can be done in the form of a dipole at the surface or line-source exciting the PC, coupling of an external Laser source or a Gaussian beam from one side, evanescent wave coupling and so on. A common scenario would be to use a waveguide coupling. Supplementary Figure 6 shows the directivity plots of an all-dielectric DLWA made from a 4 × 15-cell slab of an all-dielectric PC operating in the telecom regime. The antenna is excited with an incoming dielectric slab waveguide, as shown in the inset of Supplementary Fig. 6 , and it is shown that leaky radiation from the sides is also possible. The concept of the DLWA is introduced, which operates based on leaky-wave radiation from the interface of a PC with a Dirac-type dispersion behaviour. The DLWA has a closed stopband as well as appropriate radiation mechanisms such that it is capable of true-matched broadside radiation. The DLWA has a perfect matching, non-fluctuating leakage constant and a real Bloch impedance at and around the Γ-point. The 1D structure can be made to radiate from different sides to create narrow and directive fan beams. The 2D version of the DLWA can also yield sharp pencil beams aiming directly at broadside. With changing the frequency, the DLWA is capable of continuously scanning the beam off broadside at both forward and backward directions over a wide range of angles and without breaking up into two separate beams. DLWAs can find various applications from microwave all the way up to optical frequencies to achieve highly directive leaky-wave radiation, including radar, terahertz and optical beam-shaping, spectroscopy, free-space multiplexed optical interconnects, efficiency enhancements in opto-electronic devices and others. Design of the 1D leaky Dirac PC unit cell We begin from the unperforated (non-leaky) 2D Dirac PC of Fig. 1 as a starting point in the design towards the 1D leaky Dirac PC. Around the Dirac frequency, the Dirac PC will have an effective zero index. Therefore in the 1D PC cell of Fig. 2b , if the metallic walls of the waveguide touch the sidewalls of the unit cell (the dashed lines in Fig. 4c ), we are faced with a zero-index-filled waveguide which will be shorted. Therefore, one needs perfect magnetic conductors (PMCs) on the two sidewalls of the unit cell. This was done in ref. 3 by using mushroom-type PMC structures. An alternative simple approach is implemented here. The walls of the guide are simply extended by about λ 0 /(4 n host ) on either side of the guide, to convert the electric short into an electric open at the two sides of the PC. Therefore an open boundary condition at the two sides of the unit cell is created at the Dirac frequency allowing the two modes of interest to exist. This non-leaky 1D PC with extended sidewalls can have a closed bandgap when the Dirac-type dispersion is established due to the accidental degeneracy of its two Γ-point eigenmodes. We then introduce perforations to the unit cell to allow for leakage, leading to the 1D leaky PC unit cell of Fig. 2b . Similar sized slots were used for this purpose to make the Q of both eigenmodes finite (both radiating) and of comparable magnitude, to enable true broadside radiation as well as proper matching [22] . This, however, perturbs the PC and thus may separate the frequency of the Γ-point eigenmodes from each other, so much so as to open a bandgap in the leaky PC. To account for this impact of the slot perforations and to minimize their effects as much as possible, we then perform eigenmode simulations to tune the ‘1D leaky PC unit cell’. In this step, we adjust the leaky unit cell accordingly to again establish the Dirac dispersion in the 1D leaky PC cell. By proper adjustment of the post dimension and period, we make the Γ-point ( k x =0) eigenmodes of the leaky unit cell degenerate again. This was possible as these two eigenmodes are orthogonal and can coexist at the same frequency at the Γ-point. Thus, we arrive at a 1D leaky Dirac PC unit cell. A similar strategy can be taken for tuning the three Γ-point ( k x =0, k y =0) eigenmodes of the 2D leaky PC unit cell of Fig. 2a to become accidental degenerate, to establish the Dirac dispersion for a 2D leaky periodic structure, thus arriving at a 2D leaky Dirac PC unit cell. The eigenmode simulations of the leaky PC unit cell are carried out using the Finite Element Method eigenmode solver in Ansoft HFSS v15. Absorbing perfectly matched layer boundaries are placed in the transverse plane around the cell (at a distance away from the structure) to mimic the radiation condition. Periodic boundaries are placed in the direction of periodicity, covering the entire area and extended to also cover the relevant sides of the perfectly matched layers. Γ-point condition is applied to these periodic boundaries for the tuning stage. Hence the final stage of the design of the 1D DLWA involved tuning the filling ratio and period of the 1D leaky PC unit cell to achieve degeneracy of the two eigenmodes at the Γ-point with finite Q s. This step helps to re-establish the Dirac dispersion in the Leaky PC cell and achieve the necessary radiation conditions as in ref. 21 . We then directly cascaded N of such cells into an N-cell DLWA. The reported results for the DLWAs are using this design approach. As the reported results indicate, we readily reach a very well performing N-cell antenna, without the need for performing any other optimization on the N-cell antenna itself. Configuration of the DLWA The structure of the DLWA in Fig. 4 has a period of a =12.4 μm (in the x -direction), a substrate height of 3.9 μm (in the z -direction) and a waveguide width of 21.28 μm (in the y -direction). The dielectric rods are at the centre of each cell and have a square cross-section with dimensions 5.222 × 5.222 μm (in the x – y plane). The perforations in the top metal of the guide are slots with dimensions 8 × 1.5 μm (parallel to the x -axis) and 8 × 3 μm (parallel to the y -axis). The 19-cell antenna has a total length of 235.6 μm in the x -direction. The leaky region is connected to an incoming air-filled metallic waveguide of equal cross-section. Note that the incoming air-filled waveguide has only its fundamental TE 10 mode above cut-off. The second cut-off frequency is at 14 THz, away from the design frequency. The low dielectric constant of the host material is ε r =2.79, and the high dielectric constant of the rods is ε r =12.11, similar to ref. 15 . The choice of these PC materials can be altered based on the frequency of operation (microwaves, terahertz or optical) and availability of material/technology, losses and so on. As long as there is enough contrast between the permittivity of the rods and the host to sustain the Bloch modes of interest with no immediate spurious modes in their close vicinity in terms of frequency, the choice of materials is flexible. For instance ref. 6 demonstrated experimentally that Si and SiO 2 may be used at λ 0 =1390, nm for the rods and the host, respectively. How to cite this article: Memarian, M. et al . Dirac leaky-wave antennas for continuous beam scanning from photonic crystals. Nat. Commun. 6:5855 doi: 10.1038/ncomms6855 (2015).